A clonotypic Vγ4Jγ1/Vδ5Dδ2Jδ1 innate γδ T-cell population restricted to the CCR6+CD27−subset Here we investigate the TCR repertoire of mouse Vγ4 + γδ T cells in correlation with their developmental origin and homeostasis. By deep sequencing we identify a high frequency of straight Vδ5Dδ2Jδ1 germline rearrangements without P- and N-nucleotides within the otherwise highly diverse Trd repertoire of Vγ4 + cells. This sequence is infrequent in CCR6 − CD27 + cells, but abundant among CCR6 + CD27 − γδ T cells. Using an inducible Rag1 knock-in mouse model, we show that γδ T cells generated in the adult thymus rarely contain this germline-rearranged Vδ5Dδ2Jδ1 sequence, confirming its fetal origin. Single-cell analysis and deep sequencing of the Trg locus reveal a dominant CDR3 junctional motif that completes the TCR repertoire of invariant Vγ4 + Vδ5 + cells. In conclusion, this study identifies an innate subset of fetal thymus-derived γδ T cells with an invariant Vγ4 + Vδ5 + TCR that is restricted to the CCR6 + CD27 − subset of γδ T cells. γδ T cells use Rag -mediated V(D)J recombination to rearrange T-cell antigen receptors (TCRs) consisting of γ and δ chains. In theory, the potential junctional diversity of γδ TCRs is in the range of 10 18 , and thus several orders of magnitudes higher than that of αβ TCR or Ig rearrangements [1] . However, γδ T cells are often regarded as innate T cells that use their TCR recombination machinery to generate identical γδ TCRs of limited diversity. This perception is based on the occurrence of a few prominent γδ T-cell subsets with no or little TCR junctional diversity, in which anatomical localization and function correlate with invariant γδ TCRs [2] , [3] . Specifically, the mouse skin epidermis contains a specialized γδ T-cell population of dendritic epidermal T cells (DETCs) with a fixed TCR composed of invariant Vγ5Jγ1Cγ1 and germline-rearranged Vδ1Dδ2Jδ2 without P- or N-nucleotides (Tonegawa nomenclature) [4] , [5] . The same canonical Vδ1Dδ2Jδ2 chain is employed in combination with an invariant Vγ6Jγ1Cγ1TCR chain in interleukin (IL)-17-producing Vγ6/Vδ1 T cells. These Vγ6/Vδ1 cells were initially thought to be restricted to the uterus and the tongue [6] , but subsequently were also found in most other tissues including the lung [7] , liver [8] , dermis [9] , [10] , secondary lymphoid organs [11] and intestinal lamina propria [12] . Finally, IL-4-producing Vγ1 + γδ NKT cells with restricted Vδ6Dδ2Jδ1 junctions and semi-invariant Vγ1Jγ4Cγ4 junctions are preferentially localized in the liver and spleen [13] , [14] . In contrast, γδ T cells circulating in the blood and secondary lymphoid organs mostly contain either Vγ1 or Vγ4 rearrangements and are thought to have highly diverse TCR repertoires [3] , [15] , [16] , [17] , [18] . Recently, γδ T-cell populations grouped on the basis of the TCR γ-chain usage were included into the ImmGen transcriptome database [19] . The data suggested that γδ effector T-cell function correlated with γδ TCR usage also in Vγ4 + T cells. Fetal thymic, and to a lesser extent splenic, Vγ4 + T cells were recognized as γδ effector T cells associated with IL-17 production [19] . However, the pool of Vγ4 + T cells is heterogeneous and contains both innate cells with IL-17-producing capacity as well as cells that are biased to interferon (IFN)-γ production. These two populations can be segregated according to a CCR6 + CD27 − or CCR6 − CD27 + surface marker phenotype, respectively [20] , [21] , [22] . In addition, Vγ4 + T cells also comprise CD27 + CD45RB high cells, a subset that readily produces IFN-γ upon stimulation with IL-18 and IL-12 (ref. 23 ), similar to NK1.1 + γδ T cells [21] . Moreover, the requirements for final differentiation into effector cells may vary between γδ T-cell types depending on their ontogeny [24] . For example, it was recently proposed that Vγ4 + T cells but not Vγ6 + T cells require extrathymic maturation for imprinting of skin-homing properties and acquisition of an IL-17-producing phenotype [25] . To address the correlation of Vγ4 + TCR and Vγ4 + T-cell function in more detail, we performed a high-resolution analysis of the mouse γδ TCR repertoire. Focusing on Vγ4 + T cells, rearranged Trd and Trg loci of the respective subsets were sequenced using 454 high-throughput sequencing technology. We found striking differences in functionally different subsets of Vγ4 + T cells. Importantly, this study identifies invariant Vγ4 + Vδ5 + T cells as a novel innate T-cell population that is abundant only among CCR6 + CD27 − γδ T cells, which are known for their IL-17-producing phenotype [10] , [18] , [20] , [21] , [22] , [24] , [26] , [27] . Highly diverse Trd repertoire in Vγ1 + and Vγ4 + cells Most γδ T cells in the blood and secondary lymphoid organs display a TCR that comprises either Vγ1 or Vγ4 rearrangements. In contrast to fetal Vγ5 + DETCs or invariant Vγ6 + γδ T cells, which have a restricted TCR repertoire of very limited diversity, circulating Vγ1 + or Vγ4 + T cells are assumed to be far more polyclonal [18] . To investigate their TCR diversity in depth, we sorted these two major subsets of peripheral γδ T cells on the basis of a γδ T-cell-specific reporter fluorescence [28] and co-staining with monoclonal antibodies (mAbs) directed against their Vγ1 + or Vγ4 + TCR. Next, mRNA of these samples was amplified by rapid amplification of cDNA ends (RACE) using a gene-specific primer within the first exon of the constant gene segment of the Trd locus to amplify all rearranged VDJ combinations ( Fig. 1a ). We observed differentially biased recombination of Trd chains in Vγ1 + and Vγ4 + cells. Approximately 60% of the Trd chains from Vγ1 + samples contained a Vδ6 segment, followed by Vδ2, Vδ1, Vδ7 and Vδ12 ( Fig. 1b ). Trd chains from Vγ4 + samples contained mainly rearrangements of Vδ7 segments (~55%), followed by Vδ2, Vδ5 and Vδ6 ( Fig. 1c ). This extends but is largely consistent with prior studies based on Vδ-specific mAbs [29] . Further analysis of individual CDR3 sequences revealed a highly diverse repertoire in both Vγ1 + and Vγ4 + cells ( Supplementary Fig. 1 ). A notable exception to broad Trd polyclonality was observed only in Vδ5 rearrangements within the pool of Vγ4 + cells, where one Vδ5 + Dδ2 + Jδ1 + sequence was remarkably abundant ( Supplementary Fig. 1 ). 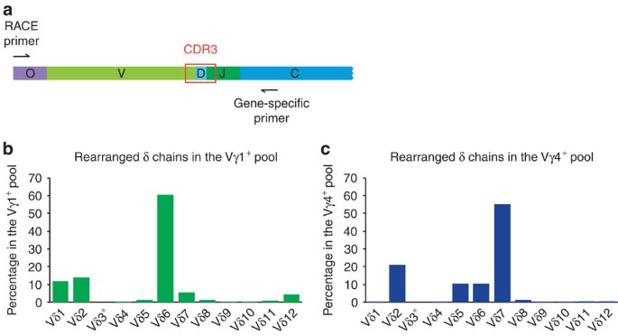Figure 1: Vδ gene segment usage among Vγ1+and Vγ4+cells from peripheral lymphoid organs. (a) Schematic presentation of a rearrangedTrdlocus and primers for RACE PCR (O: SMARTer anchor oligonucleotide; V: variable, D: diversity, J: joining and C: constant gene segments). (b,c) Results of RACE PCR product sequencing. Bars indicate proportion of in-frame rearrangements of Vδ gene segments within the purified Vγ1+or Vγ4+cells pooled from the pLN and spleen of threeTcrdH2BeGFPmice. (*: Vδ3 is a pseudogene). For each Vγ pool, at least 22,000 in-frame sequences were analysed. Data are representative of two independent experiments that gave similar results. Figure 1: Vδ gene segment usage among Vγ1 + and Vγ4 + cells from peripheral lymphoid organs. ( a ) Schematic presentation of a rearranged Trd locus and primers for RACE PCR (O: SMARTer anchor oligonucleotide; V: variable, D: diversity, J: joining and C: constant gene segments). ( b , c ) Results of RACE PCR product sequencing. Bars indicate proportion of in-frame rearrangements of Vδ gene segments within the purified Vγ1 + or Vγ4 + cells pooled from the pLN and spleen of three TcrdH2BeGFP mice. (*: Vδ3 is a pseudogene). For each Vγ pool, at least 22,000 in-frame sequences were analysed. Data are representative of two independent experiments that gave similar results. Full size image Abundant Vδ5Dδ2Jδ1 rearrangements in Vγ4 + cells In order to further investigate the occurrence of abundant Vδ5Dδ2Jδ1 sequence in γδ T cells, we applied primers that specifically amplified CDR3 regions located between Vδ5 and Jδ1 segments ( Fig. 2a ). With this independent approach, we confirmed the data obtained by RACE analysis. On the amino-acid level, ~30% of Vδ5 + Trd sequences in Vγ4 + cells isolated from secondary lymphoid organs showed a unique arrangement of Vδ5, Dδ2 and Jδ1 segments, whereas this combination was absent in Vγ1 + T cells, and represented less than 0.3% of Vδ5 + Trd sequences in intestinal Vγ7 + cells ( Fig. 2b ). Importantly, the Vδ5, Dδ2 and Jδ1 segments were directly rearranged without P- and N-nucleotides (hereafter called germline rearrangements) in more than 95% of these canonical Trd sequences, while other nucleotide sequences coding for the same CDR3 amino-acid sequence were uncommon ( Table 1 ). Next, we hypothesized that these canonical Vδ5Dδ2Jδ1 sequences originated from Vγ4 + γδ T cells that had developed in the fetal thymus, similar to the invariant Trd chains found in Vγ5 + DETCs and in Vγ6 + γδ T cells. Their TCRs share canonical N-nucleotide-lacking Vδ1Dδ2Jδ2 rearrangements [4] , [5] , [6] . To this end, we sequenced the Vδ5 repertoire of Vγ4 + γδ T cells sorted from either wild-type TcrdH2BeGFP control mice (wt) or from Indu- Rag1 mice [30] crossed with TcrdH2BeGFP mice. In the latter, deficient V(D)J recombination had been restored in the adult stage by tamoxifen-induced cre recombinase expression. Only ~1% of the canonical Vδ5Dδ2Jδ1 rearrangements were found when only adult γδ T-cell development had been possible in Indu- Rag1 mice as compared with control Vγ4 + γδ T cells with more than 30% of such sequences ( Fig. 2c ). These results suggest that the large majority of canonical Vγ4 + /Vδ5Dδ2Jδ1 + γδ T cells are generated early in ontogeny, presumably in the embryonic thymus. 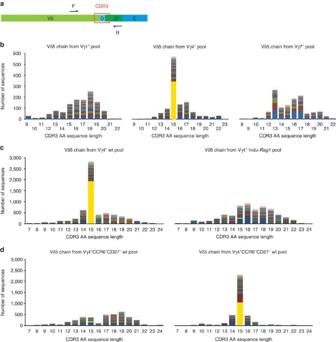Figure 2: One Vδ5Dδ2Jδ1 sequence is dominant in CCR6+CD27−Vγ4+T cells. (a) Schematic presentation of a rearrangedTrdlocus showing the position of representative primers used for amplification of variableTrdregions between Vδ5 and Jδ1, F: forward primer, R: reverse primer. (b) CDR3 amino-acid sequence length distribution and composition for in-frame rearrangements of Vδ5–Jδ1 chain in Vγ1+T cells (left panel), and Vγ4+T cells (middle panel) isolated from a pool of pLN and spleen, or Vγ7+intestinal IELs (right panel), of threeTcrdH2BeGFPmice in each subset. (c) In-frame rearrangements of Vδ5–Jδ1 chains in Vγ4+T cells pooled from the pLN and spleen of fourTcrdH2BeGFPmice (wt; left panel) or four tamoxifen-induced Indu-Rag1xTcrdH2BeGFPmice (right panel). Genomic DNA from 10,000 Vγ4+T cells was used as template. For each subset, 5,870 sequences were analysed. (d) In-frame rearrangements of Vδ5–Jδ1 chains in CCR6−CD27+(left panel) versus CCR6+CD27−(right panel) Vγ4+T cells pooled from the pLN and spleen of threeTcrdH2BeGFPmice. cDNA from 4,800 CCR6−CD27+or CCR6+CD27−Vγ4+cells was used as template. For each subset, 3,552 sequences were analysed. Individual in-frame-rearranged CDR3 amino-acid sequences are separated by colours. Data are representative of at least two independent experiments that gave similar results. Figure 2: One Vδ5Dδ2Jδ1 sequence is dominant in CCR6 + CD27 − Vγ4 + T cells. ( a ) Schematic presentation of a rearranged Trd locus showing the position of representative primers used for amplification of variable Trd regions between Vδ5 and Jδ1, F: forward primer, R: reverse primer. ( b ) CDR3 amino-acid sequence length distribution and composition for in-frame rearrangements of Vδ5–Jδ1 chain in Vγ1 + T cells (left panel), and Vγ4 + T cells (middle panel) isolated from a pool of pLN and spleen, or Vγ7 + intestinal IELs (right panel), of three TcrdH2BeGFP mice in each subset. ( c ) In-frame rearrangements of Vδ5–Jδ1 chains in Vγ4 + T cells pooled from the pLN and spleen of four TcrdH2BeGFP mice (wt; left panel) or four tamoxifen-induced Indu- Rag1 x TcrdH2BeGFP mice (right panel). Genomic DNA from 10,000 Vγ4 + T cells was used as template. For each subset, 5,870 sequences were analysed. ( d ) In-frame rearrangements of Vδ5–Jδ1 chains in CCR6 − CD27 + (left panel) versus CCR6 + CD27 − (right panel) Vγ4 + T cells pooled from the pLN and spleen of three TcrdH2BeGFP mice. cDNA from 4,800 CCR6 − CD27 + or CCR6 + CD27 − Vγ4 + cells was used as template. For each subset, 3,552 sequences were analysed. Individual in-frame-rearranged CDR3 amino-acid sequences are separated by colours. Data are representative of at least two independent experiments that gave similar results. Full size image Table 1 Most frequent Vδ5 CDR3 nucleotide sequences that encode the canonical V δ 5 amino-acid sequence. Full size table Canonical rearrangements in CCR6 + CD27 − γδ T cells Next, we tested whether Vγ4 + cells with canonical Vδ5Dδ2Jδ1 rearrangements were contributing to the pool of IL-17-producing Vγ4 + γδ T cells, as these were recently discovered to develop exclusively before birth and subsequently persist in adult mice as self-renewing, long-lived cells [11] . Such IL-17-producing effector γδ T cells are contained within a population of γδ T cells identified by a CCR6 + CD27 − surface marker phenotype [20] , [21] , [22] . Therefore, we sorted Vγ4 + T cells from peripheral lymph nodes (pLNs) and spleen of adult TcrdH2BeGFP mice into CCR6 − CD27 + and CCR6 + CD27 − subsets, sequenced their Trd loci and compared them with each other. Clearly, canonical Vδ5Dδ2Jδ1 rearrangements were highly enriched in the CCR6 + CD27 − subset ( Fig. 2d ). Thereby, the corresponding CDR3 amino-acid motif ASGYIGGIRATDKLV from CCR6 + CD27 − Vγ4 + T cells was principally but not exclusively encoded by Vδ5Dδ2Jδ1 rearrangements unmodified by P- or N-nucleotides ( Fig. 3 ). Together, these results suggest that CCR6 + CD27 − Vγ4 + T cells have a distinct TCR repertoire that comprises canonical Vδ5Dδ2Jδ1 + γδ T cells. The data further support the hypothesis that IL-17-producing CCR6 + CD27 − Vγ4 + T cells are principally generated within a functional wave of embryonic γδ T-cell development [11] , [18] . 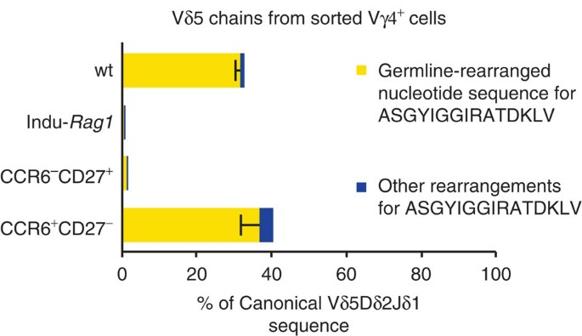Figure 3: Frequency of a canonical Vδ5Dδ2Jδ1 CDR3 sequence. Bar graphs show percentages of the canonical CDR3 amino-acid sequence ASGYIGGIRATDKLV among in-frame Vδ5 sequences derived from the indicated Vγ4+T-cell populations. Yellow bars represent dominant rearrangements of germline-Vδ5, -Dδ2 and -Jδ1 segments without P- and N-nucleotides. Error bars show s.e.m. Blue bars represent the sum of all other nucleotide sequences coding for ASGYIGGIRATDKLV. Data are pooled from two independent experiments that gave similar results. Figure 3: Frequency of a canonical Vδ5Dδ2Jδ1 CDR3 sequence. Bar graphs show percentages of the canonical CDR3 amino-acid sequence ASGYIGGIRATDKLV among in-frame Vδ5 sequences derived from the indicated Vγ4 + T-cell populations. Yellow bars represent dominant rearrangements of germline-Vδ5, -Dδ2 and -Jδ1 segments without P- and N-nucleotides. Error bars show s.e.m. Blue bars represent the sum of all other nucleotide sequences coding for ASGYIGGIRATDKLV. Data are pooled from two independent experiments that gave similar results. Full size image Ontogeny and organ distribution of Vδ5Dδ2Jδ1 + T cells To further explore the potential fetal thymic origin of canonical Vδ5Dδ2Jδ1 + Vγ4 + T cells, we sorted Vγ4 + T cells derived from the thymus at different stages during ontogeny and sequenced the Trd repertoire of Vδ5–Jδ1 amplicons ( Fig. 4a ). The invariant Vδ5Dδ2Jδ1 sequence was already abundant in the fetal thymic Trd repertoire of Vγ4 + T cells on embryonic day 18 (E18, 15% of all Vδ5 sequences), but also persisted in juvenile (11–17%) or adult thymi (7% at 4 months; Fig. 4a and Supplementary Fig. 2 ). These data further support the hypothesis that IL-17-producing γδ T cells, in particular with the invariant Vδ5Dδ2Jδ1 clonotype, are already generated in the fetal thymus, but later persist as resident cells in the juvenile and adult thymus [11] , [24] . Moreover, these findings are consistent with a previous ontogeny study as described in (ref. 31 ). However, invariant Vδ5Dδ2Jδ1 + T cells were even more abundant in peripheral lymphoid organs than in the thymus, suggesting peripheral homeostatic expansion of the subset. Notably, invariant Vδ5Dδ2Jδ1 + Trd sequences made up 43% of all Vδ5 sequences of Vγ4 + T cells in pLNs and 27% in the spleen ( Fig. 4b ). Because TCR repertoire as well as the developmental requirements of Vγ4 + T cells vary along with location [25] , we investigated different peripheral anatomical sites separately. By deep sequencing of Vδ5–Jδ1 amplicons we examined the TCR repertoire of Vγ4 + T cells derived from other organs including the lung, skin and liver ( Fig. 4b and Supplementary Fig. 3 ). It turned out that the invariant Vδ5Dδ2Jδ1 sequence also dominated the Trd repertoire of Vγ4 + T cells in peripheral tissues such as the skin (27%), lung (15%) and liver (25%), albeit to a lesser extent than in pLNs. Across all samples derived from the pLN and spleen, the Vδ5Dδ2Jδ1 clonotype made up ~35% of the Vδ5 repertoire in Vγ4 + T cells. Since ~10% of Vγ4 + T cells used the Vδ5 segment (as shown by RACE analyses in Fig. 1 ), these constitute 3.5% clonotypic cells of all Vγ4 + T cells. Thus, with Vγ4 + T cells making up to 50% of all γδ T cells derived from the pLN [32] , the actual rate of clonotypic invariant Vδ5Dδ2Jδ1 + γδ T cells is 1.5–2% among all γδ T cells. This remarkably high frequency is in the range of invariant IL-17A-producing Vγ6Vδ1 + T cells that constitute 2–4% among all γδ T cells in secondary lymphoid organs [33] , [34] . Nevertheless, only moderate expansion of this subset in peripheral tissues as compared with the thymus underlines their genuine innate nature. 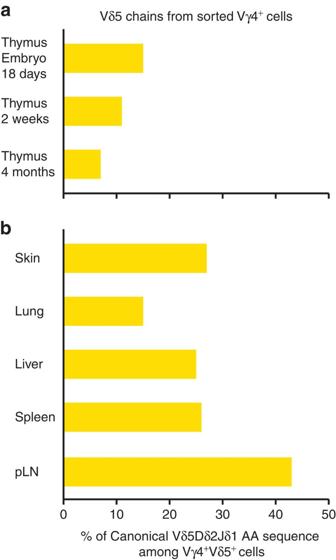Figure 4: Frequency of a canonical Vδ5Dδ2Jδ1 CDR3 sequence in thymus ontogeny and in peripheral tissues. Bar graphs show percentages of the canonical CDR3 amino-acid sequence ASGYIGGIRATDKLV among in-frame Vδ5 sequences derived from the indicated fluorescence-activated cell sorting-sorted Vγ4+T-cell populations. (a) Frequency of the canonical CDR3 sequence in the thymus of day E18 old embryos, 2-week-old pups and 4-month-old adult mice. (b) Frequency of canonical CDR3 sequence in the skin, lung, liver, spleen and pLN. Data represent eight individual samples from one 454-sequencing run. Figure 4: Frequency of a canonical Vδ5Dδ2Jδ1 CDR3 sequence in thymus ontogeny and in peripheral tissues. Bar graphs show percentages of the canonical CDR3 amino-acid sequence ASGYIGGIRATDKLV among in-frame Vδ5 sequences derived from the indicated fluorescence-activated cell sorting-sorted Vγ4 + T-cell populations. ( a ) Frequency of the canonical CDR3 sequence in the thymus of day E18 old embryos, 2-week-old pups and 4-month-old adult mice. ( b ) Frequency of canonical CDR3 sequence in the skin, lung, liver, spleen and pLN. Data represent eight individual samples from one 454-sequencing run. Full size image Decreased TCR diversity in CCR6 + CD27 − Vγ4 + T cells Next, we asked whether TCR diversity in noninvariant Vγ4 + Vδ5 + T cells among the CCR6 + CD27 − subset was also different to CCR6 − CD27 + Vγ4 + T cells ( Fig. 5 ). Within an equally sized pool of in-frame amino-acid sequences obtained from both populations, CCR6 − CD27 + Vγ4 + T cells had a higher proportion of unique Vδ5 rearrangements that were present only once in the tested sample (singletons), while CCR6 + CD27 − Vγ4 + T cells showed fewer singletons ( Fig. 5a ). Consequently, samples from CCR6 + CD27 − Vγ4 + T cells contained a higher frequency of sequences that were detected several times. In Fig. 5b , in which all sequences are represented according to their actual frequency among all sequences, such clones were considered as expanded (1–1.99%) or highly expanded (≥ 2%). To quantify the TCR diversity of the respective two γδ T-cell subsets, we calculated the effective number of sequences using the Shannon index, which considers the number of observed individual sequences as well their abundance in the repertoire [35] , [36] . It turned out that the CCR6 + CD27 − subset was three times less diverse than CCR6 − CD27 + cells, and still two times less diverse when the dominant canonical Vδ5Dδ2Jδ1 sequence was excluded from the equation ( Fig. 5c ). Qualitatively, we observed essentially no overlapping Vδ5 sequences between two independently analysed samples of CCR6 − CD27 + Vγ4 + cells. The only exception was the canonical sequence that was found repeatedly, albeit at low frequency ( Fig. 5d , left panel). In contrast, two independent samples of CCR6 + CD27 − Vγ4 + T cells showed an overlap of 29 Trd sequences, beside the canonical Vδ5Dδ2Jδ1 sequence ( Fig. 5d , right panel). Accordingly, the similarity of two independent samples, calculated as the Morisita–Horn index, was low (0.003) for CCR6 − CD27 + and high (0.889) for CCR6 + CD27 − Vγ4 + T cells. In conclusion, CCR6 + CD27 − Vγ4 + T cells, which are known for their IL-17-production capacity, display TCR repertoires of limited diversity and a considerable TCR sequence overlap between independent samples derived from individual mice. This is consistent with the view that these cells develop as a population of prewired innate effector cells with limited TCR diversity in the fetal thymus to persist and expand after birth. 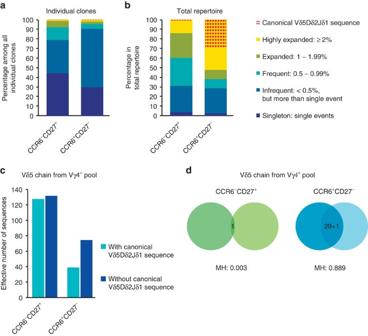Figure 5: TCR diversity of CCR6−CD27+versus CCR6+CD27−Vγ4+cells. (a) Proportion of 309 individual sequences of CCR6−CD27+Vγ4+cells, or 276 individual sequences of CCR6+CD27−Vγ4+cells, among 3,552 Vδ5 sequences of each subset. Each individual sequence is counted only once regardless of abundance. (b) Proportion of total sequences from the same pool asa, considering the abundance. Fora,b, data shown are from one representative of two independent experiments. (c) Diversity measured as ‘effective number of sequences’ (eto the power of the Shannon index) for the same data set of 3,552 CDR3 amino-acid sequences in each subset, including the canonical sequence (light blue), or after eliminating the canonical sequence from the repertoires (dark blue). (d) Venn diagrams display overlap between the 100 most frequent CDR3 amino-acid sequences in similar populations from two independent experiments. Numbers indicate overlapping individual sequences. Similarity between the repertoires from two independent experiments was calculated using the Morisita–Horn index (MH). The MH index reveals the degree of similarity by analysing individual sequences considering their frequency among the total repertoire, scoring from 0 for completely dissimilar subsets to 1 for identical subsets. Figure 5: TCR diversity of CCR6 − CD27 + versus CCR6 + CD27 − Vγ4 + cells. ( a ) Proportion of 309 individual sequences of CCR6 − CD27 + Vγ4 + cells, or 276 individual sequences of CCR6 + CD27 − Vγ4 + cells, among 3,552 Vδ5 sequences of each subset. Each individual sequence is counted only once regardless of abundance. ( b ) Proportion of total sequences from the same pool as a , considering the abundance. For a , b , data shown are from one representative of two independent experiments. ( c ) Diversity measured as ‘effective number of sequences’ ( e to the power of the Shannon index) for the same data set of 3,552 CDR3 amino-acid sequences in each subset, including the canonical sequence (light blue), or after eliminating the canonical sequence from the repertoires (dark blue). ( d ) Venn diagrams display overlap between the 100 most frequent CDR3 amino-acid sequences in similar populations from two independent experiments. Numbers indicate overlapping individual sequences. Similarity between the repertoires from two independent experiments was calculated using the Morisita–Horn index (MH). The MH index reveals the degree of similarity by analysing individual sequences considering their frequency among the total repertoire, scoring from 0 for completely dissimilar subsets to 1 for identical subsets. Full size image The corresponding Vγ4 repertoire To complement the Trd repertoires, we next determined the respective Vγ4 repertoires of sorted Vγ4 + T-cell populations. Sequencing was performed using a Vγ4-specific primer in combination with a consensus primer amplifying Jγ1, Jγ2 and Jγ3 ( Fig. 6 ). Consistent with previous findings [2] , [37] , overall diversity of the rearranged Trg loci was lower than at Trd loci, and more than 99% of Vγ4 rearrangements involved Jγ1. Analysis of CDR3 amino-acid sequence length distribution and composition of Vγ4 chain repertoires demonstrated an expanded Vγ4 motif, SYGXYSSGFHKV. Notably, this dominant motif was abundant in Vγ4 + T cells derived from wt and Indu- Rag1 mice ( Fig. 6a ) as well as in CCR6 − CD27 + and CCR6 + CD27 − Vγ4 + T cells ( Fig. 6b ). This is in contrast to our findings for the canonical Vδ5Dδ2Jδ1 Trd locus rearrangement, which was exclusively abundant in fetal thymus-derived CCR6 + CD27 − γδ T cells. Nevertheless, the Vγ4 repertoire of the IL-17-producing CCR6 + CD27 − subset was even more focused towards the SYGXYSSGFHKV consensus CDR3 sequence than CCR6 − CD27 + Vγ4 + T cells ( Fig. 6b ). Among all Vγ4 chain sequences analysed, a leucine residue was most frequently found at the variable position X of this CDR3 motif, followed by serine, arginine, proline and subsequently all other amino acids ( Fig. 6c ). While a stop codon within the germline Vγ4 segment precludes true germline rearrangements, the two most frequent nucleotide sequences coding for SYGLYSSGFHKV were still rather germline-like as they both lacked N-nucleotides ( Table 2 ). Together, these two sequences accounted for one-third of all in-frame sequences obtained from the CCR6 + CD27 − subset of Vγ4 + T cells ( Fig. 6d ). In conclusion, sequence analyses of the corresponding Vγ4 repertoire is consistent with the view that rearrangement at the γ and δ TCR loci is differentially controlled. Furthermore, the presence of the semi-invariant Vγ4 sequences also in CCR6 − CD27 + Vγ4 + T cells and in T cells from Indu- Rag1 mice would alone not be sufficient for any potential positive selection of IL-17-producing CCR6 + CD27 − subset of Vγ4 + T cells. 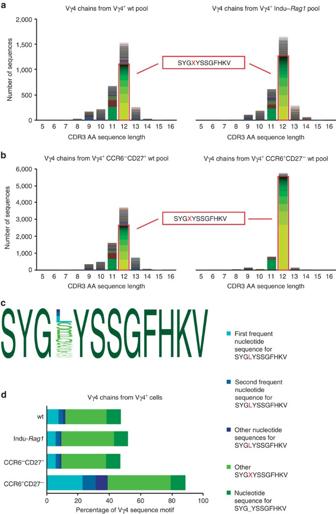Figure 6: A frequent motif in the Vγ4 repertoire. (a,b) CDR3 amino-acid sequence length distribution and composition of in-frame-rearranged Vγ4 chains in (a) Vγ4+γδ T cells pooled from the pLN and spleen of fourTcrdH2BeGFPor four tamoxifen-induced Indu-Rag1×TcrdH2BeGFPmice; 10,000 Vγ4+cells and 2,892 in-frame sequences each. (b) CCR6−CD27+or CCR6+CD27−Vγ4+T cells isolated from the pooled pLN and spleen of threeTcrdH2BeGFPmice; 12,000 Vγ4+cells and 6,888 in-frame sequences each. Individual in-frame-rearranged CDR3 amino-acid sequences are separated by colours. Sequences containing the SYGXYSSGFHKV motif are shown in green tones within a red box, and the sequence SYG_YSSGFHKV (lacking X) with 11 amino acids is also shown in green. Data are representatives of three independent experiments. (c) Graphical representation of multiple sequence alignment for the frequent Vγ4 amino-acid motif, SYGXYSSGFHKV, inspired byhttp://weblogo.berkeley.edu. (d) Percentage of the most frequent CDR3 sequence, SYGLYSSGFHKV, and the proportion of its related nucleotide sequences (in blue tone), along with percentage of other nucleotide sequences containing the SYGXYSSGFHKV motif (in light green), and the sequences for SYG_YSSGFHKV (in dark green), within all in-frame Vγ4 sequences of the indicated populations. Data are representative of two independent experiments that gave similar results. Figure 6: A frequent motif in the Vγ4 repertoire. ( a , b ) CDR3 amino-acid sequence length distribution and composition of in-frame-rearranged Vγ4 chains in ( a ) Vγ4 + γδ T cells pooled from the pLN and spleen of four TcrdH2BeGFP or four tamoxifen-induced Indu- Rag1 × TcrdH2BeGFP mice; 10,000 Vγ4 + cells and 2,892 in-frame sequences each. ( b ) CCR6 − CD27 + or CCR6 + CD27 − Vγ4 + T cells isolated from the pooled pLN and spleen of three TcrdH2BeGFP mice; 12,000 Vγ4 + cells and 6,888 in-frame sequences each. Individual in-frame-rearranged CDR3 amino-acid sequences are separated by colours. Sequences containing the SYGXYSSGFHKV motif are shown in green tones within a red box, and the sequence SYG_YSSGFHKV (lacking X) with 11 amino acids is also shown in green. Data are representatives of three independent experiments. ( c ) Graphical representation of multiple sequence alignment for the frequent Vγ4 amino-acid motif, SYGXYSSGFHKV, inspired by http://weblogo.berkeley.edu . ( d ) Percentage of the most frequent CDR3 sequence, SYGLYSSGFHKV, and the proportion of its related nucleotide sequences (in blue tone), along with percentage of other nucleotide sequences containing the SYGXYSSGFHKV motif (in light green), and the sequences for SYG_YSSGFHKV (in dark green), within all in-frame Vγ4 sequences of the indicated populations. Data are representative of two independent experiments that gave similar results. Full size image Table 2 Most frequent V γ 4 CDR3 nucleotide sequences that encode the V γ 4 amino-acid sequence SYG L YSSGFHKV. Full size table Invariant Vδ5Dδ2Jδ1 chains pair with a canonical Vγ4 chain Finally, we sought to identify the corresponding TCR γ and TCR δ chain pairs that constituted the TCR heterodimer of IL-17-producing CCR6 + CD27 − Vγ4 + T cells. To this end, we performed single-cell PCR from cDNA of sorted Vγ4 + CCR6 + CD27 − cells. Of 20 individual T cells with Vδ5Dδ2Jδ1 Trd germline rearrangement, 7 had Trg rearrangements coding for the most frequent Vγ4 CDR3 sequence SYG L YSSGFHKV, 12 displayed other variations of the SYG X YSSGFHKV motif and one clone showed a shorter version of this CDR3, namely SYG_YSSGFHKV ( Table 3 ). Together, these results suggest that the pool of fetal thymus-derived IL-17-producing γδ T cells of the CCR6 + lineage contains a population of invariant Vγ4 + cells with a TCR composed of a germline-rearranged Vδ5Dδ2Jδ1 chain and a canonical Vγ4Jγ1 chain motif. Table 3 Single-cell analysis of 20 V γ 4 chains pairing with the canonical V δ 5D δ 2J δ 1 chain. Full size table This study focused on the correlation between TCR sequence and effector phenotype in Vγ4 + T cells, which constitute a heterogenic population of mouse γδ T cells. It comprised high-throughput generation of hundreds of thousands of sequences of rearranged Trg and Trd genes and constitutes, to our knowledge, the first deep-sequencing report on Trd genes in any species as well as on mouse Trg genes. In general, our results clearly support the view that diversity of rearranged Trd loci is much higher than for their Trg counterparts. In particular, the mouse Vγ4 repertoire contained predominant expanded sequences that were shared between individual mice. These findings are consistent with prior deep-sequencing studies of the human TRG repertoire [38] , [39] , which described a limited diversity in the TRG repertoire. There [38] , the TRG repertoire of peripheral blood γδ T cells from three independent donors was dominated by canonical Vγ9JγP sequences. In sharp contrast to the Trg locus, our study showed that the Trd repertoire was highly diverse in sorted Vγ4 + and Vγ1 + T cells from peripheral lymphoid organs. Most importantly, we revealed a novel invariant subset of innate γδ T cells, with a TCR composed of a canonical Vγ4Jγ1 motif paired with germline-rearranged Vδ5Dδ2Jδ1. This invariant TCR rearrangement might have evolved under selective pressure for simple and efficient modular recombination without any N- or P-nucleotides of the respective loci yielding a useful invariant TCR. Furthermore, it is conceivable that the canonical CDR3δ loop might interact with putative TCR ligands autonomously and uncoupled from the variable CDR3γ. Such mode of γδ TCR–ligand interaction would be reminiscent of γδ TCR recognition of the nonclassical major histocompatibility complex class I molecules T10 and T22 (refs 40 , 41 ). While relatively short CDR3δ chains can bind to model antigens such as phycoerythrin (PE) or Cyanine Dye Cy3 (Cy-3) haptens only in combination with a suitable CDR3γ partner, a relatively long CDR3δ loop such as the canonical Vδ5Dδ2Jδ1 rearrangement (15 AA according to the international ImMunoGeneTics information system®) may be indeed be indicative of CDR3γ-independent ligand binding. In addition, the novel invariant Vγ4 + Vδ5 + T-cell population shares several decisive features with three other prominent invariant γδ T-cell subsets in mice, which are Vγ5 DETCs, Vγ6 + Vδ1 + cells and semi-invariant Vγ1 + Vδ6 + NKT cells and likewise fetal liver-derived human Vγ9 + Vδ2 + cells [42] . First, all of these populations contain straight germline rearrangements of invariant canonical TCRs without nontemplated N-nucleotides. Second, they are of fetal or at least perinatal origin. These two features, canonical germline rearrangements and exclusive development in the fetal thymus, define such γδ T-cell populations as genuine innate T cells. Invariant Vγ4 + Vδ5 + T cells were remarkably abundant in every sample of Vγ4 + T cells sorted by a CCR6 + CD27 − surface phenotype associated with IL-17-producing capacity and basically absent in CCR6 − CD27 + Vγ4 + T cells. Importantly, these results were very reproducible and consistent regardless of whether independent samples were derived from genomic DNA or cDNA and whether these were analysed by either RACE or Vδ5-specific primers. Thus, the canonical Vγ4 + Vδ5 + TCR classifies a hitherto unrecognized conserved subset of innate and presumably IL-17-producing Vγ4 + T cells. Notably, invariant Vγ4 + Vδ5 + T cells are actually abundant in peripheral lymphoid organs in the same magnitude as IL-17-producing Vγ6 + Vδ1 + cells [33] , [34] . In future studies, it will be interesting to compare the common and discrete functions of these two invariant γδ T-cell subsets that are likely innate ‘natural’ IL-17A-producers. Interestingly, identical Vδ5Dδ2Jδ1 germline rearrangements had 24 years ago been designated as BID, for BALB/c invariant delta [43] . These Trd germline rearrangements were described as frequent in lungs and lymph nodes of mice with a BALB/c genetic background, but are absent in mice with a C57BL/6 genetic background [43] . However, BID chains were later found to be generated also in C57BL/6 fetal thymocytes at levels similar to those detected in BALB/c mice [44] . Hence, it was concluded that the presence of BID among resident pulmonary lymphocytes of BALB/c and of BALB/c × C57BL/6 F1 mice but not in C57BL/6 mice was because of positive selection and peripheral expansion [44] . Yet, in our study, γδ T cells bearing BID, that is, Vδ5Dδ2Jδ1 germline rearrangements, turned out to be an abundant innate Vγ4 + T-cell population in C57BL/6 mice. It is currently unclear, however highly relevant for future work, why the C57BL/6 mice of our study and the C57BL/6 mice of the Basel Institute used as negative controls for the original BID description in 1990 would differ in this respect. It is tempting to speculate that specific genetic variations are responsible for differential selection and peripheral expansion processes. This might provide a remarkable analogy to the seminal observation that a substrain of inbred FVB mice was uniquely depleted of invariant Vγ5 + DETCs [45] , which led to the discovery of the DETC-selecting determinant Skint-1 (refs 46 , 47 ). In any case, identification of potential cognate ligands of the invariant TCRs from canonical Vγ4 + Vδ5 + T cells, as well as Vγ5 DETCs, Vγ6 + Vδ1 + cells and semi-invariant Vγ1 + Vδ6 + NKT cells, has highest priority. Formerly suggested candidates for the selection of invariant Vγ4 + Vδ5 + T cells, called BID + cells, included the murine heat-shock protein 60 (ref. 48 ) and a potential self-ligand that correlates with the presence of the endogenous murine leukaemia virus Mpmv -30 (ref. 49 ). Furthermore, it needs to be determined in future studies whether innate invariant Vγ4 + Vδ5 + T cells accumulate or expand in response to inflammatory stimuli and during bacterial infection as reported for invariant Vγ6 + Vδ1 + cells [12] , [50] , [51] , [52] . The null hypothesis, however, is that no specific antigen is required for selection and development of canonical innate Vγ4 + Vδ5 + T cells. This would be consistent with the hypothesis that the capacity to produce IL-17 cytokines is prewired in a subset of fetal T-cell precursors before and is independent of TCR rearrangement [11] . In addition, there is considerable evidence that positively selecting TCR-triggering in immature fetal γδ T-cell precursors induces differentiation towards the potential to produce IFN-γ while suppressing the IL-17-associated factors Sox13 , Sox4 and Rorc [32] , [53] , [54] , [55] . Thus, if TCR-specific selection of invariant Vγ4 + Vδ5 + T cells occurred during thymic development, they would, in contrast to our observations, be rather expected to adopt a CCR6 − CD27 + phenotype with the potential to produce IFN-γ. In conclusion, we establish a novel truly innate γδ T-cell subset of invariant Vγ4 + Vδ5 + T cells, which is confined to presumably IL-17-producing CCR6 − CD27 + T cells. Future studies addressing the specific physiological functions of these cells within the pLNs and within tissues such as the lung, skin and liver will advance the understanding of innate lymphocyte and γδ T-cell biology. Mice All mice used throughout the study were on a C57BL/6 genetic background. C57BL/6- TcrdH2BeGFP mice were generated at the Centre d’Immunologie de Marseille-Luminy [28] and C57BL/6-Indu- Rag1 mice were a kind gift from Siggi Weiß [30] . Indu- Rag1 mice were crossed to TcrdH2BeGFP to obtain tamoxifen-inducible Indu- Rag1 × TcrdH2BeGFP mice [11] at the animal facilities of the Helmholtz Centre for Infection Research, Braunschweig. C57BL/6- TcrdH2BeGFP and C57BL/6 wild-type control mice were bred and maintained under specific pathogen-free conditions at the animal facility of the Hannover Medical School, and used at 8–14 weeks of age (16 weeks in case of Indu- Rag1 × TcrdH2BeGFP mice) if not otherwise stated in the figure legends. Animal experiments were carried out according to the institutional guidelines approved by the local government. This study was performed in accordance with the German Animal Welfare Law and with the European Communities Council Directive 86/609/EEC for the protection of animals used for experimental purposes. Cell isolation and cell sorting pLNs and spleens were mashed, filtered through 50-μM nylon meshes and washed with PBS/3% fetal calf serum. Spleen cells were treated with erythrocyte-lysis buffer before mixing with lymph node cells as described previously [56] . The liver and lung were cut into small pieces and digested with 0.5 mg ml −1 Collagenase D and 0.025 mg ml −1 DNAse-1. The digestion was stopped by adding EDTA to a final concentration of 20 mM. For the isolation of skin lymphocytes, an area of the back was shaved, the skin was removed and cut into pieces and digested with 0.5-mg ml −1 Liberase and 0.025 mg ml −1 DNAse-1. Digestion was carried out for 45 min at 37 °C and was stopped by adding EDTA to a final concentration of 40 mM. Digested organs were meshed through a 40-μm Cellstrainer. Lung lymphocytes were separated using Lympholyte M. Liver and skin lymphocytes were separated with density gradient centrifugation using Percoll gradients. MAbs against TCR Vγ4 (clone UC3-10A6, PE-conjugated, 1:200) were purchased from Biolegend or produced in rat hybridoma cell lines (clone 49.2-9, Cy5-conjugated, 1:100). Antibody against TCR Vγ1 (clone 2.11, PE-conjugated, 1:100) was purchased from Biolegend and antibody against TCR Vγ7 (clone F2.67, Cy5-conjugated, 1:50) produced in rat hybridoma cell lines. Antibodies against TCR β (clone H57-597, PE-Cy7-conjugated, 1:200) and CD27 (clone LG.3A10, PerCP/Cy5.5-conjugated, 1:200) were obtained from Biolegend. Antibodies against CD196 (CCR6; clone 140706, Alexa Fluor 647-conjugated, 1:100) were purchased from BD Biosciences. Cell suspensions were treated with FcR block (clone 2.4G2) before 20-min staining with mAbs. Antibody-labelled cell populations were sorted for high-throughput sequencing through the FACSAria IIu flow cytometer (Becton Dickinson). In experiments designed to compare two populations, we always sorted the same amount of cells as a starting population to be able to quantify TCR diversities. Likewise, single cells were sorted into 96-well plates for single-cell PCR by MoFlo or XDP flow cytometer (Beckman-Coulter). The first rows of the plates were left empty as negative controls. Nucleic acid isolation For isolation of genomic DNA, sort-purified cell fractions were resuspended in PCR lysis buffer (10 mM Tris (pH 8.4), 50 mM KCl, 2 mM MgCl 2 , 0.5% Nonidet P-40, 0.5% Tween-20, 400 μg ml −1 proteinase K) at 500 cells μl −1 and incubated overnight at 50 °C. The proteinase K was inactivated at 95 °C for 10 min. This protocol was adapted from refs 56 , 57 , 58 . Up to 20 μl of the DNA samples were used directly for PCR. Total RNA was isolated from sorted cell populations using the RNeasy Mini Kit (QIAGEN) and was reverse-transcribed with Superscript III (Invitrogen) using Random Primers (Invitrogen). RACE To generate unbiased template libraries of rearranged CDR3 regions of the Trd locus, anchor sequence-containing cDNA template was synthesized using the SMARTer RACE cDNA Amplification Kit (Clontech) according to the manufacturer. RACE PCR was performed with a gene-specific primer located in the Cδ gene segment (5′- CGAATTCCACAATCTTCTTG -3′) and an anchor sequence-specific primer recommended in the kit. Gene-specific PCR PCR was performed to generate amplicon libraries of rearranged TCR sequences. Gene-specific primers (Vγ4: 5′- TGCAACCCCTACCCATATTTTCT -3′ in combination with a consensus primer amplifying Jγ1, 2 and 3: 5′- GTTCCTTCTGCAAATACCTTGTGA -3′ or Vδ5: 5′- AGCACAGCAAGGCCAACAGAACCTT -3′ in combination with Jδ1: 5′- TTGGTTCCACAGTCACTTGGGTTCC -3′). Either genomic DNA or cDNA were amplified using 0.375 μM of each forward and reverse primers, 50 μM of each dNTP, 1.5 mM MgCl 2 and 2.5 U Taq DNA Polymerase (invitrogen) in a 50-μl reaction. Amplifications were performed at 94 °C for 4 min, followed by 35 cycles consisting of 30 s at 94 °C, 30 s at 59 °C and 20 s at 72 °C, and finally a single incubation at 72 °C for 5 min. High-throughput sequencing Forward and reverse PCR primers for deep-sequencing contained at their 5′ ends the respective 454 universal adaptor sequences and multiplex identifier (MID) nucleotides. PCR products were purified using gel extraction with the QIAquick Gel Extraction kit (QIAGEN) and was quantified with Qubit fluorometer (Invitrogen) using the Quant-iT dsDNA HS Assay kit (Invitrogen). Amplicons were processed with the emPCR—Lib-A SV kit (GS FLX Titanium series; Roche) according to the manufacturer to sequence on 454 Genome Sequencer FLX system (Roche). Productive rearrangements and CDR3α regions were defined by comparing nucleotide sequences to the reference sequences from IMGT, the international ImMunoGeneTics information system ( http://www.imgt.org ) [59] . Rearrangements were analysed and CDR3α regions were defined using IMGT/HighV-QUEST [60] . Single-cell PCR For single-cell PCR, CCR6 + CD27 − Vγ4 + single cells were sorted directly into 96 wells. We reverse-transcribed RNA from each sort-purified cell to cDNA, and used it as a template to amplify corresponding γ and δ TCR chains. Single cells sorted in 6-μl PBS were immediately frozen on dry ice and transferred to −80 °C. Frozen cells were lysed by heating to 65 °C for 2 min and were cooled to 4 °C. RNA transcription and a first round of PCR were sequentially performed in one reaction using the OneStep RT–PCR kit (QIAGEN) according to the manufacturer with some modifications. A combination of specific5′- primer pair for Vγ4 chain (Vγ4 outer: 5′- ASCAAGAGATGAGACTGCACAAAT -3′ in combination with Jγ1, 2 and 3: 5′- GTTCCTTCTGCAAATACCTTGTGA -3′) and Vδ5 chain (Vδ5 outer: 5′- TGCGGATTCTCCAAACCCAGATTTA -3′ in combination with Jδ1: 5′- TTGGTTCCACAGTCACTTGGGTTCC -3′) was used for this multiplex reaction. For a 25-μl reaction, the components were as following: 1 × buffer, 400 μM of each dNTP, 0.4 μM of each primer and 1-μl OneStep RT–PCR Enzyme mix. Reverse transcription was performed for 30 min at 50 °C and was directly followed by amplification. PCR activation was initiated at 95 °C for 15 min, before 30 cycles, consisting of 30 s at 94 °C, 30 s at 65 °C and 60 s at 72 °C, and finally a single incubation at 72 °C for 10 min. Next, second rounds of PCR with seminested primers (Vγ4: 5′- TGCAACCCCTACCCATATTTTCT -3′ and Vδ5 inner: 5′- TAGGGACGACACTAGTTCCCATGAT -3′) were separately performed for Vγ4 and Vδ5 chains. For this, 0.2 μl from the first PCR products were used as template in a 20-μl reaction. The PCR fragments were amplified using 0.5 unit AmpliTaq Gold DNA polymerase (Applied Biosystems) in combination with GeneAmp 1 × PCR puffer II, 2 mM MgCl 2 , 0.25 mM of each dNTP and 0.3 μM of each primer. After 10 cycles, samples positive for Vγ4 and Vδ5 were detected using agarose gel electrophoresis. After additional 20 cycles of PCR, gel-extracted (QIAGEN) PCR products of Vγ4 and Vδ5 chains from each cell were separately cloned in pCR4-TOPO vector through the TOPO TA Cloning Kit for sequencing (Invitrogen). These plasmid vectors were isolated via the QIAprep kit (QIAGEN) and sequenced by GATC Biotech (Germany). Sequence analysis First, fna files generated by 454 high-throughput sequencing were converted and partitioned into separate FASTA files using MIDs and gene-specific primer sequence identifiers. Next, these files were uploaded to HighV-QUEST, an online tool available on the IMGT website [59] , and compared with the IMGT data base. Analysed txt files returned from IMGT were further processed with Excel to segregate productive and unproductive TCR rearrangements to quantify and merge similar sequences and for further statistical analysis. Via specifically selecting only in-frame productive TCR rearrangements, sequences that contained insertions and deletions from the 454 platform were routinely excluded. Shannon indices were calculated using Vegan R package (2.14.0). Venn diagrams were produced with VennMaster (0.37.5; ref. 61 ). All raw sequence data were uploaded to the NCBI Sequence Read Archive under the SRP accession number SRP050364 . How to cite this article: Kashani, E. et al . A clonotypic Vγ4Jγ1/Vδ5Dδ2Jδ1 innate γδ T-cell population restricted to the CCR6 + CD27 − subset. Nat. Commun. 6:6477 doi: 10.1038/ncomms7477 (2015).